Rio1 promotes rDNA stability and downregulates RNA polymerase I to ensure rDNA segregation The conserved protein kinase Rio1 localizes to the cytoplasm and nucleus of eukaryotic cells. While the roles of Rio1 in the cytoplasm are well characterized, its nuclear function remains unknown. Here we show that nuclear Rio1 promotes rDNA array stability and segregation in Saccharomyces cerevisiae . During rDNA replication in S phase, Rio1 downregulates RNA polymerase I (PolI) and recruits the histone deacetylase Sir2. Both interventions ensure rDNA copy-number homeostasis and prevent the formation of extrachromosomal rDNA circles, which are linked to accelerated ageing in yeast. During anaphase, Rio1 downregulates PolI by targeting its subunit Rpa43, causing PolI to dissociate from the rDNA. By stimulating the processing of PolI-generated transcripts at the rDNA, Rio1 allows for rDNA condensation and segregation in late anaphase. These events finalize the genome transmission process. We identify Rio1 as an essential nucleolar housekeeper that integrates rDNA replication and segregation with ribosome biogenesis. At anaphase onset, the replicated chromosomes separate and then segregate along the mitotic spindle into the daughter cells. In the budding yeast Saccharomyces cerevisiae , the locus containing the genes that encode the ribosomal RNAs (rDNA) segregates after the rest of the genome, in late anaphase [1] , [2] , [3] , [4] . The rDNA locus exists as a tandem-repeat array comprising ∼ 150 rDNA units containing the 35S and 5S genes, which are transcribed by RNA polymerase I (PolI) and PolIII, respectively. Processing of the 35S pre-rRNA generates 5.8S, 18S and 25S rRNA that, together with the 5S rRNA, become the catalytic backbones of each ribosome [5] , [6] . Only in anaphase does yeast repress rDNA transcription [4] , which allows the sister rDNA loci to condensate and segregate. PolI downregulation in anaphase is mediated by the Cdc14 phosphatase acting on PolI subunit Rpa43 (ref. 4 ), resulting in PolI dissociating from the 35S rDNA. The removal of PolI and the local resolution of its transcripts allow the condensin complex to bind. The latter compacts the rDNA array and recruits the DNA decatenating enzyme topoisomerase II (refs 1 , 3 , 4 , 7 ) resulting in the physical separation and subsequent segregation of the sister rDNA loci. S. cerevisiae Rio1 belongs to the atypical RIO protein kinase family whose members lack the activation loop and substrate recognition domain present in canonical eukaryotic protein kinases [8] , [9] , [10] , [11] . Noteworthy, the RIO kinases may act especially as ATPases as they exhibit <0.1% kinase activity in vitro [12] , [13] , [14] . Cytoplasmic Rio1 contributes to pre-40S ribosome biogenesis by promoting 20S pre-rRNA maturation and by stimulating the recycling of trans-acting factors at the pre-40S subunit, both in yeast [12] , [15] , [16] , [17] , [18] and human cells [19] , [20] . Roles in the nucleus are unknown for any RIO member, either in yeast or eukaryotes beyond. Using S. cerevisiae , we now describe the first activities of Rio1 in the nucleus. Foremost, Rio1 downregulates PolI transcription through the cell cycle. In G1, Rio1 additionally promotes pre-rRNA processing to ensure a timely commencement of the cell cycle. In S phase, besides downregulating PolI, Rio1 also recruits the histone deacetylase Sir2 to ensure rDNA repeat-number stability. In anaphase, the downregulation of PolI by Rio1 and its activation of pre-rRNA processing drive rDNA condensation and segregation. Cells lacking nuclear Rio1 activity suffer from a delayed cell cycle entry, fragmented nucleolus, an expanded rDNA array, extrachromosomal rDNA circles (ERCs) and an inability to segregate rDNA. We identify Rio1 as an essential nucleolar housekeeper of rDNA integrity and transmission, and as an upstream regulator of ribosome biogenesis. Rio1 localizes dynamically to rDNA during the cell cycle Previous work showed that substituting conserved catalytic residue D244E in the Rio1 kinase domain provoked plasmid loss in S. cerevisiae [21] , suggesting an involvement of Rio1 in DNA replication and/or segregation. To examine this possibility, we imaged Rio1, labeled with green fluorescent protein (Rio1-GFP), in exponentially growing S. cerevisiae cells. We identified the protein both in the cytoplasm (consistent with its documented involvement in 20S pre-rRNA maturation [15] and pre-40S ribosome trans-factor recycling [12] , [17] , [18] ), and in the nucleus ( Fig. 1a ). As the intranuclear localization of Rio1 could not be easily determined, we isolated the nuclei from exponentially grown yeast, crosslinked and then spread them on glass slides. Immunofluorescence (IF) microscopy with an anti-Rio1 antibody revealed that Rio1 was highly enriched at the nucleolus (co-localized with nucleolar marker Nop1; Fig. 1b ), the subnuclear compartment that is organized around the rDNA array ( Supplementary Fig. 1 ). However, Rio1 signal intensities were heterogeneous across the nuclei suggesting a cell cycle-dependent localization. To probe this observation further, 6myc-Rio1 cells were arrested in G1 with α-factor and then synchronously released into the cell cycle. Samples were taken during cell cycle progression, the nuclei were isolated, spread and analysed by anti-myc IF imaging ( Fig. 1c,d ). We observed that Rio1 was highly enriched at the nucleolus in G1. Rio1 signals then decreased by half through S phase. In metaphase, the nucleoli contained very low amounts of Rio1, whereas at anaphase onset Rio1 became actively re-recruited to the nucleolus, reaching levels similar to those measured in G1 ( Fig. 1c,d and Supplementary Fig. 2a ). Low amounts of Rio1 were detectable in the nucleus (beyond the nucleolus), especially in S phase ( Fig. 1d ). Using chromatin immunoprecipitation (ChIP) analysis, we next probed to which sites Rio1 localized at the rDNA. 6myc-Rio1 cells were arrested in G1, S phase, metaphase and anaphase (via use of α-factor, hydroxyurea, nocodazole and the cdc15-2 allele, respectively). The rDNA sequences that were enriched with immunoprecipitated Rio1 were identified by real-time quantitative PCR (RT–qPCR) analysis using probes covering the rDNA unit. While the 6myc-Rio1 signals were distributed homogeneously across the rDNA in G1 and metaphase cells, we found the kinase to be enriched at the 35S rDNA promoter and gene sequence (probes 4 and 5) in S phase and anaphase (coloured lines in Fig. 1e ). However, the averaged values obtained with the five probes (black bars in Fig. 1e ) confirmed the Rio1 localization dynamics observed by imaging of the spread nuclei. 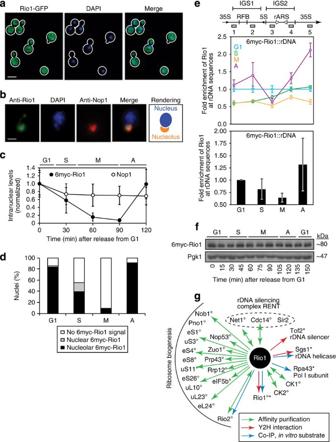Figure 1: Rio1 localizes to the rDNA in a dynamic, cell cycle stage-dependent manner. (a) Fluorescence microscopy image of DAPI-stained exponentially growing yeast cells endogenously expressing Rio1-GFP. Scale bar, 5 μm. (b) Indirect IF image of Rio1 (anti-Rio1) and nucleolar marker Nop1 (anti-Nop1) in a spread nucleus isolated from a G1 cell. Scale bar, 5 μm. (c) Nuclear 6myc-Rio1 and Nop1 levels (normalized to Nop1 concentrations in G1) measured from IF images (anti-myc, anti-Nop1) of spread nuclei isolated from cells progressing through the cell cycle. Error bars, s.d.’s,n=50 per time point. (d) Intranuclear distribution of 6myc-Rio1 established from IF images of spread nuclei isolated from cells synchronously progressing through the cell cycle (from the experiment depicted inc).n=50 Per time point. (e) 6myc-Rio1 protein levels at the rDNA as quantified by ChIP–qPCR analysis of cells arrested in G1, S phase, metaphase (M) or anaphase (A). Positions of the real-time qPCR probes along the rDNA unit are indicated (1–5). IGS, intergenic spacer region; RFB, replication fork barrier; rARS, origin of replication; 5S and 35S, genes encoding 5S and 35S rRNA, respectively. The upper plot shows the data obtained with each probe per cell cycle stage (each data point corresponds to the probe indicated above). Error bars, s.d.’s.n=3. The lower plot shows the averages of the values obtained with the five probes. (f) Western blot of endogenous 6myc-Rio1 protein levels (anti-myc) through the cell cycle (Pgk1=loading control). (g) The Rio1 interactome. Rio1 interactors reported in the literature [°]25and identified in this study [*]). Figure 1: Rio1 localizes to the rDNA in a dynamic, cell cycle stage-dependent manner. ( a ) Fluorescence microscopy image of DAPI-stained exponentially growing yeast cells endogenously expressing Rio1-GFP. Scale bar, 5 μm. ( b ) Indirect IF image of Rio1 (anti-Rio1) and nucleolar marker Nop1 (anti-Nop1) in a spread nucleus isolated from a G1 cell. Scale bar, 5 μm. ( c ) Nuclear 6myc-Rio1 and Nop1 levels (normalized to Nop1 concentrations in G1) measured from IF images (anti-myc, anti-Nop1) of spread nuclei isolated from cells progressing through the cell cycle. Error bars, s.d.’s, n =50 per time point. ( d ) Intranuclear distribution of 6myc-Rio1 established from IF images of spread nuclei isolated from cells synchronously progressing through the cell cycle (from the experiment depicted in c ). n =50 Per time point. ( e ) 6myc-Rio1 protein levels at the rDNA as quantified by ChIP–qPCR analysis of cells arrested in G1, S phase, metaphase (M) or anaphase (A). Positions of the real-time qPCR probes along the rDNA unit are indicated (1–5). IGS, intergenic spacer region; RFB, replication fork barrier; rARS, origin of replication; 5S and 35S, genes encoding 5S and 35S rRNA, respectively. The upper plot shows the data obtained with each probe per cell cycle stage (each data point corresponds to the probe indicated above). Error bars, s.d.’s. n =3. The lower plot shows the averages of the values obtained with the five probes. ( f ) Western blot of endogenous 6myc-Rio1 protein levels (anti-myc) through the cell cycle (Pgk1=loading control). ( g ) The Rio1 interactome. Rio1 interactors reported in the literature [°] [25] and identified in this study [*]). Full size image A previous report indicated that Rio1, overexpressed from the P GAL10 promoter, becomes degraded in S phase, suggesting Rio1 stability is cell cycle regulated [22] . However, our western blot analyses of yeast endogenously expressing Rio1 showed that its protein levels do not change through the cell cycle ( Fig. 1f ). Hence, the observed dynamic localization of Rio1 may reflect changes in its affinity for nucleolar factors and/or its active import–export from the nucleus. Rio1 shuttling between the nucleus and cytoplasm was evidenced previously by its intranuclear accumulation in an exportin mutant [16] . Besides its localization, a role for Rio1 at the rDNA was indicated by its recent co-purification with the phosphatase Cdc14 and its inhibitor Cfi1 (ref. 23 ), which together with the histone deacetylase Sir2 form the rDNA-silencing complex RENT [24] ( Fig. 1g ). Our own yeast two-hybrid screens that used Rio1 as the bait ( Supplementary Fig. 2b ) identified as interactors the rDNA helicase Sgs1 (confirmed by co-immunoprecipitation from yeast whole-cell extract; Supplementary Fig. 2c ), the rDNA-silencing protein Tof2 and Rio1 itself ( Supplementary Fig. 2b ). These findings extend the current Rio1 protein-interaction map that mostly comprises ribosome biogenesis factors [25] ( Fig. 1g ). Distinct sets of nucleolar proteins recruit Rio1 While the 150-unit repeat nature of the rDNA array satisfies yeast’s huge demand for ribosomes [26] , its configuration makes rDNA highly vulnerable to genetic instability during rDNA replication [27] , [28] . Although the replication fork moves bi-directionally from the rARS, the leftward-moving replisome is halted at the replication fork barrier site (RFB) to prevent it from colliding with PolI, transcribing the 35S rDNA sequence in rightward direction. Such a collision would generate incomplete 35S rRNA transcripts and produce double-strand breaks in the 35S unit. However, the replisome held at the RFB may collapse, resulting in the exposure of single-strand rDNA, progressing into a double-strand break. Double-strand DNA breaks are repaired by homologous recombination. For a correct repair to occur, the sister rDNA loci must be aligned. If not, homologous recombination will result in an expansion or contraction of the rDNA array and in the formation of ERCs [27] , [28] , anomalies that have been linked to a shortened lifespan in yeast [29] , [30] . Various proteins contribute to sister rDNA alignment and faithful recombination, as described in Supplementary Fig. 1 . They include Fob1, Tof2, RENT (Cfi1, Cdc14, Sir2), Sgs1, and the monopolin, cohesin and condensin complexes. To determine the basis for the cell cycle-stage-dependent localization of Rio1 to the rDNA, we probed Rio1 recruitment by IF analysis of spread nuclei isolated from mutants lacking one of the above rDNA factors. Cells were released from G1 or S phase (a sir2Δ mutant does not respond to α-factor) and then tracked through the cell cycle by analysis of spindle morphology (anti-Tub1 IF) and DNA content (fluorescence-activated cell sorting, FACS) ( Supplementary Fig. 3 ). In short, we found that Rio1 localization to rDNA in interphase depended on Fob1, Sgs1, Sir2 and Cdc14, while its anaphase recruitment required Fob1, Sgs1, monopolin and condensin ( Fig. 2a,b and Supplementary Fig. 4a ). Rio1 thus localizes to the rDNA at different cell cycle stages via distinct rDNA factors (summarized in Fig. 2c ). The observed changes in Rio1 recruitment in the mutant backgrounds were not due to alterations in Rio1 expression or stability, as western blot analyses showed that Rio1 protein levels remained constant through the cell cycle in all of the mutants tested ( Supplementary Fig. 4b ). Noteworthy, the phosphatase Cdc14 is kept inactive in the nucleolus from G1 through metaphase by its inhibitor Cfi1 (ref. 31 ) and becomes released (activated) at anaphase entry. However, when we inactivated and delocalized Cdc14 in G1 ( cdc14-3 mutant at the non-permissive temperature), we observed a marked reduction in Rio1 levels at interphase nucleoli and, in parallel, a distribution of the kinase throughout the nucleus ( Fig. 2b ). A constitutive release of Cdc14 instigated by removing Cfi1 ( cfi1Δ ) confirmed this observation. Hence, albeit anchored in the nucleolus, Cdc14 serves at least to recruit Rio1 to interphase rDNA. 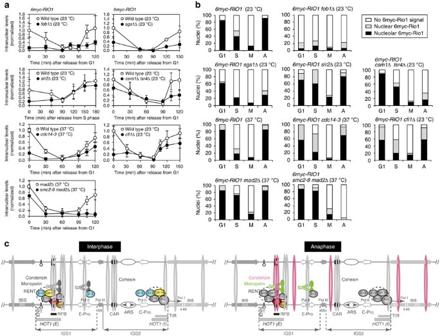Figure 2: Distinct sets of nucleolar proteins recruit Rio1 to interphase and anaphase rDNA. (a) Nuclear levels of 6myc-Rio1 through the cell cycle of strains mutated in a single rDNA regulator as determined by quantitative IF imaging (anti-myc) of spread nuclei. Signals are normalized to the 6myc-Rio1 levels measured in the wild-type control strains in G1. Error bars, s.d.’s.n=50 Per time point. (b) Intranuclear distribution of 6myc-Rio1 in specific cell cycle stages (n=50) as probed by IF imaging of spread nuclei isolated from the cells ina. (c) Graphic representation of the rDNA factors (coloured) that recruit Rio1 to rDNA in interphase (left) and anaphase (right). Figure 2: Distinct sets of nucleolar proteins recruit Rio1 to interphase and anaphase rDNA. ( a ) Nuclear levels of 6myc-Rio1 through the cell cycle of strains mutated in a single rDNA regulator as determined by quantitative IF imaging (anti-myc) of spread nuclei. Signals are normalized to the 6myc-Rio1 levels measured in the wild-type control strains in G1. Error bars, s.d.’s. n =50 Per time point. ( b ) Intranuclear distribution of 6myc-Rio1 in specific cell cycle stages ( n =50) as probed by IF imaging of spread nuclei isolated from the cells in a . ( c ) Graphic representation of the rDNA factors (coloured) that recruit Rio1 to rDNA in interphase (left) and anaphase (right). Full size image Characterization of a Rio1 nuclear depletion mutant To study Rio1 activity at the rDNA, we wished to inducibly remove the kinase from the nucleus only. Based on the observation that Rio1 shuttles between the nucleus and the cytoplasm [16] , we figured that conditionally removing its C-terminal tail containing a putative nuclear localization signal (NLS; Supplementary Fig. 5a ) would prevent truncated Rio1 from entering the nucleus. Rio1 present in the nucleus at the moment of truncation should still be able to exit from the nucleus as its putative nuclear exit signal localizes at the outer edge of the RIO domain ( Fig. 3a and Supplementary Fig. 5b ). To allow for conditional truncation, we cloned the Tobacco Etch Virus (TEV) Protease with a C-terminal NLS under control of the galactose-inducible P GAL10 promoter on a high-copy plasmid (next named p P GAL10 - TEV Protease ; Supplementary Fig. 5c ). Next, we introduced a TEV Protease cleavage site just upstream of the NLS in 6myc-Rio1 (next referred to as 6myc-Rio1 TEV ; Fig. 3a ). To confirm the TEV Protease-induced cleavage of 6myc-Rio1 TEV , we grew the 6myc-rio1 TEV strains carrying p P GAL10 - TEV Protease or the empty p P GAL10 vector (negative control) in 2% raffinose medium and then treated the cells for 1 h with 2% galactose. TEV Protease expression led to the removal of 6myc-Rio1’s C-terminal 78 residues ( Fig. 3b ), as indicated by anti-myc western blot analysis. Within the hour, truncated 6myc-Rio1 TEV had also become depleted from the nucleus as shown by IF microscopy of spread nuclei ( Fig. 3c ) and whole cells ( Fig. 3d ). Whereas 6myc-Rio1 TEV was no longer detected in the nucleus, its signals could still be observed and quantified in the cytoplasm ( Fig. 3d ). When plated on 2% galactose medium, the mutant strain died, indicating that the C-terminal region of Rio1 is essential for viability, in agreement with previous observations [12] . Importantly, overexpressing the TEV Protease in wild-type yeast did not affect viability ( Fig. 4a ). 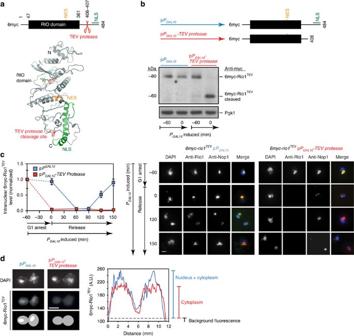Figure 3: Depletion of Rio1 from the nucleus. (a) The Rio1 nuclear depletion construct. To-scale representation and computational model of the 6myc-Rio1TEVprotein. The RIO domain, the putative nuclear export signal (NES), the putative NLS and the TEV Protease cleavage site (introduced between E406 and E407) are indicated. The model of full-length 6myc-Rio1TEVbound to ATP and manganese was generated with Phyre2 (http://www.sbg.bio.ic.ac.uk/phyre2) based on the structure ofA. fulgidusRio1 (PDB 1ZTH)45. (b) Ectopic expression of the TEV Protease truncates the 6myc-Rio1TEVprotein at its C-terminus. Top: To-scale representation and western blot (anti-myc) of full-length and truncated 6myc-Rio1TEVproteins in6myc-rio1TEVpPGAL10(blue) and6myc-rio1TEVpPGAL10-TEV Protease(red) cells before and afterPGAL10induction with 2% galactose (Pgk1, loading control). (c) Intranuclear 6myc-Rio1TEVlevels in cells lacking (blue) or expressing (red) TEV Protease, quantified from IF images (anti-myc) of spread nuclei. Both strains were grown in 2% raffinose medium and arrested in G1.PGAL10was induced (1 h, 2% galactose), and the cells then released into the cell cycle (2% galactose medium, 150 min).n=50 Per time point. Error bars, s.d.’s. Representative images are shown on the right. Scale bar, 5 μm. (d) IF images of 6myc-Rio1TEV(anti-myc) in anaphase-arrestedcdc15-2yeast cells that lack (left, blue) or express (right, red) TEV Protease (DAPI=DNA). Scale bar, 5 μm. Fluorescence levels were quantified along the horizontal axes. Figure 3: Depletion of Rio1 from the nucleus. ( a ) The Rio1 nuclear depletion construct. To-scale representation and computational model of the 6myc-Rio1 TEV protein. The RIO domain, the putative nuclear export signal (NES), the putative NLS and the TEV Protease cleavage site (introduced between E406 and E407) are indicated. The model of full-length 6myc-Rio1 TEV bound to ATP and manganese was generated with Phyre2 ( http://www.sbg.bio.ic.ac.uk/phyre2 ) based on the structure of A. fulgidus Rio1 (PDB 1ZTH) [45] . ( b ) Ectopic expression of the TEV Protease truncates the 6myc-Rio1 TEV protein at its C-terminus. Top: To-scale representation and western blot (anti-myc) of full-length and truncated 6myc-Rio1 TEV proteins in 6myc-rio1 TEV p P GAL10 (blue) and 6myc-rio1 TEV p P GAL10 -TEV Protease (red) cells before and after P GAL10 induction with 2% galactose (Pgk1, loading control). ( c ) Intranuclear 6myc-Rio1 TEV levels in cells lacking (blue) or expressing (red) TEV Protease, quantified from IF images (anti-myc) of spread nuclei. Both strains were grown in 2% raffinose medium and arrested in G1. P GAL10 was induced (1 h, 2% galactose), and the cells then released into the cell cycle (2% galactose medium, 150 min). n =50 Per time point. Error bars, s.d.’s. Representative images are shown on the right. Scale bar, 5 μm. ( d ) IF images of 6myc-Rio1 TEV (anti-myc) in anaphase-arrested cdc15-2 yeast cells that lack (left, blue) or express (right, red) TEV Protease (DAPI=DNA). Scale bar, 5 μm. Fluorescence levels were quantified along the horizontal axes. 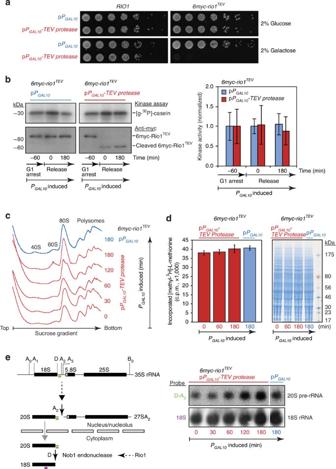Figure 4: Functional characterization of the Rio1 nuclear depletion mutant. (a) Growth of theRIO1and6myc-rio1TEVstrains carrying pPGAL10(blue) or pPGAL10-TEV Protease(red) on glucose and galactose media (23 °C). (b)In vitrokinase activity analysis of full-length or truncated 6myc-Rio1TEVisolated from yeast lacking or expressing TEV Protease, respectively. The reaction contained [γ-32P]ATP and dephosphorylated casein, as the substrate. Left; top: [γ-32P]-phosphorylated casein visualized radiographically; bottom: western blots (anti-myc) of full-length or truncated 6myc-Rio1TEV. The indicated times (min) are relative to the release from G1. Right: 6myc-Rio1TEVkinase activity normalized to the activity measured 1 h beforePGAL10induction.n=3. Error bars, s.d.’s. (c) Ribosome profiles of6myc-rio1TEVpPGAL10(blue) and6myc-rio1TEVpPGAL10-TEV Protease(red) strains. Samples were taken at the indicated time points and the cell extracts fractionated by 5–45% sucrose gradient ultracentrifugation. The 254-nm absorption profiles measured along the gradients are shown. (d) Cells depleted of nuclear Rio1 activity are not affected in protein neo-synthesis.6myc-rio1TEVpPGAL10(blue) and6myc-rio1TEVpPGAL10-TEV Proteasecells (red) were grown in 2% raffinose medium and then treated with 2% galactose. The cells were provided (20 min) with [methyl-3H]-L-methionine and its incorporation in nascent proteins quantified (scintillation counts) at the indicated time points. The numbers represent average values.n=3. Error bars=s.d’s. The extracted proteins were run in parallel on a Nu-PAGE gradient gel and then Coomassie stained, confirming that equal protein amounts were analysed for [methyl-3H]-L-methionine incorporation. (e) Northern blots of total RNA isolated from6myc-rio1TEVpPGAL10(blue) and6myc-rio1TEVpPGAL10-TEV Proteasecells (red) (from experiment ind). Positions of the D-A2(green) and 18S (purple) northern probes hybridizing with 20S pre-rRNA and 18S rRNA are indicated in the sketch on the left. Full size image Figure 4: Functional characterization of the Rio1 nuclear depletion mutant. ( a ) Growth of the RIO1 and 6myc-rio1 TEV strains carrying p P GAL10 (blue) or p P GAL10 -TEV Protease (red) on glucose and galactose media (23 °C). ( b ) In vitro kinase activity analysis of full-length or truncated 6myc-Rio1 TEV isolated from yeast lacking or expressing TEV Protease, respectively. The reaction contained [γ- 32 P]ATP and dephosphorylated casein, as the substrate. Left; top: [γ- 32 P]-phosphorylated casein visualized radiographically; bottom: western blots (anti-myc) of full-length or truncated 6myc-Rio1 TEV . The indicated times (min) are relative to the release from G1. Right: 6myc-Rio1 TEV kinase activity normalized to the activity measured 1 h before P GAL10 induction. n =3. Error bars, s.d.’s. ( c ) Ribosome profiles of 6myc-rio1 TEV p P GAL10 (blue) and 6myc-rio1 TEV p P GAL10 -TEV Protease (red) strains. Samples were taken at the indicated time points and the cell extracts fractionated by 5–45% sucrose gradient ultracentrifugation. The 254-nm absorption profiles measured along the gradients are shown. ( d ) Cells depleted of nuclear Rio1 activity are not affected in protein neo-synthesis. 6myc-rio1 TEV p P GAL10 (blue) and 6myc-rio1 TEV p P GAL10 -TEV Protease cells (red) were grown in 2% raffinose medium and then treated with 2% galactose. The cells were provided (20 min) with [methyl- 3 H]- L -methionine and its incorporation in nascent proteins quantified (scintillation counts) at the indicated time points. The numbers represent average values. n =3. Error bars=s.d’s. The extracted proteins were run in parallel on a Nu-PAGE gradient gel and then Coomassie stained, confirming that equal protein amounts were analysed for [methyl- 3 H]- L -methionine incorporation. ( e ) Northern blots of total RNA isolated from 6myc-rio1 TEV p P GAL10 (blue) and 6myc-rio1 TEV p P GAL10 -TEV Protease cells (red) (from experiment in d ). Positions of the D-A 2 (green) and 18S (purple) northern probes hybridizing with 20S pre-rRNA and 18S rRNA are indicated in the sketch on the left. Full size image To determine whether truncated Rio1 remains a functioning kinase, we measured the kinase activity of full-length and cleaved 6myc-Rio1 TEV . We synchronized the 6myc-rio1 TEV p P GAL10 -TEV Protease and 6myc-rio1 TEV p P GAL10 strains in G1 and induced TEV Protease expression with 2% galactose (1 h) while keeping the cells arrested in G1. Next, we released the cells in 2% galactose medium and took samples 1 h before, upon and 3 h after the release. Western blot analysis confirmed the C-terminal truncation of 6myc-Rio1 TEV in the strain expressing TEV Protease ( Fig. 4b ). Full-length and truncated 6myc-Rio1 TEV were then immunopurified (anti-myc beads) and their activity assayed on dephosphorylated casein [21] . The measured kinase activities were identical ( Fig. 4b ), confirming an earlier report that recombinant Rio1 lacking a similar C-terminal region is still active as a kinase in vitro [22] . To exclude a possible contribution from casein kinases CK1 and CK2, shown to co-purify with full-length Rio1 (refs 12 , 22 ) and with Rio1 lacking its C-terminal 46 residues [9] , the assay was repeated in the presence of CK1 and CK2 inhibitors. While the overall kinase activity decreased, we measured no differences between the kinase activities of full-length and truncated 6myc-Rio1 TEV ( Supplementary Fig. 6a ). The C terminus of Rio1 was previously shown to be necessary for cytoplasmic Rio1 to bind to the pre-40S ribosome and for promoting 20S pre-rRNA maturation [12] . As such, we examined whether truncated 6myc-Rio1 TEV could still mediate these functions within the 3-h time frame during which we phenotype the mutant cells (see further down). Specifically, we probed ribosome biogenesis, protein translation and 20S pre-rRNA to 18S rRNA maturation. Whole-cell extracts from exponentially grown 6myc-rio1 TEV p P GAL10 -TEV Protease and 6myc- rio1 TEV p P GAL10 strains were collected at different time points (0–3 h) after P GAL10 induction. The extracts were fractionated by 5–45% sucrose gradient ultracentrifugation and their nucleic acid profiles were recorded at 254 nm. We observed a subtle decrease in 40S subunits levels (and concomitant increase in 60S levels) at the latest time points in the cells depleted of nuclear Rio1 ( Fig. 4c ). The ribosome (80S) and polysome profiles of both strains were basically identical suggesting similar mRNA translation capacities. We confirmed this conclusion as pulse labelling of the mutant and control cultures with [methyl- 3 H]-L-methionine revealed no difference in the amount of radiolabelled methionine that was incorporated in the neo-synthesized proteins ( Fig. 4d ). Next, we probed cytoplasmic 20S pre-rRNA maturation at pre-40S particles via northern blot analysis. In good agreement with our slight decrease in 40S levels, we observed a mild 20S pre-rRNA to 18S rRNA processing defect ( Fig. 4e ). Because our data show that during the short time frame of one cell cycle (3 h), the cytoplasmic activity of truncated 6myc-Rio1 TEV is not markedly affected, we used this mutant to study how activities at the rDNA are affected in yeast depleted of nuclear Rio1. Rio1 promotes rDNA stability and segregation To phenotype the Rio1 nuclear exclusion mutant, we first analysed its progression through the cell cycle. Compared with the control cells, yeast depleted of nuclear Rio1 consistently showed a 15–20-min delay in cell cycle commencement at START (G1/S transition; orange triangles in Fig. 5a ), whereas progression through the subsequent cell cycle stages was not affected. Importantly, overproduction of the TEV Protease in a wild-type strain did not delay cell cycle initiation ( Supplementary Fig. 6b ). IF microscopy of spread nuclei revealed nucleolar fragmentation in the absence of Rio1 ( Fig. 5b ), an anomaly that is indicative of rDNA instability. To probe this phenotype further, we grew the 6myc- rio1 TEV p P GAL10 - TEV Protease and 6myc- rio1 TEV p P GAL10 strains for eight divisions in 2% galactose medium. Electrophoretic analysis of their DNA content followed by Southern blot analysis with a 25S rDNA probe [32] revealed ERCs and an expanded rDNA array, as in a sir2Δ mutant (positive control; Fig. 5c ), known to contain 200–300 rDNA units [33] . Homologous recombinations underlaid these rDNA-instability phenotypes as GFP-labelled recombination mediator Rad52 formed fluorescent foci at the nucleolar periphery, the area where rDNA recombination takes place [34] ( Fig. 5d ). Despite the rDNA hyper-recombination events, progression through S phase was not delayed ( Fig. 5a ) and the DNA damage checkpoint kinase Rad53 not activated/phosphorylated [35] ( Fig. 5e ). Importantly, the cells depleted of nuclear Rio1 were DNA checkpoint proficient as they arrested in S phase with phosphorylated Rad53 upon treatment with hydroxyurea ( Fig. 5f and Supplementary Fig. 6c ). 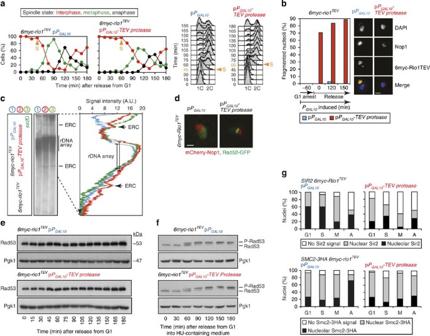Figure 5: Rio1 promotes timely cell cycle commencement and rDNA stability. (a)6myc-rio1TEVpPGAL10(blue) and6myc-rio1TEVpPGAL10-TEV Protease(red) cells were arrested in G1 (2% raffinose).PGAL10was then induced (1 h, 2% galactose) and the cells released into the cell cycle (2% galactose medium). Cells were tracked by analysis of spindle morphology (anti-Tub1 IF;n=200 cells per time point) and DNA content (FACS). The orange arrows indicate S phase. (b) Percentage of6myc-rio1TEVpPGAL10(blue) and6myc-rio1TEVpPGAL10-TEV Protease(red) cells, released from G1, with fragmented nucleoli (Nop1=nucleolar marker), as established by IF imaging analysis of spread nuclei (anti-myc, anti-Nop1).n=50 Per time point. Representative IF images are shown on the right. Scale bar, 5 μm. (c) Left: Southern blot (anti-25S) of total DNA isolated from6myc-rio1TEVpPGAL10(blue),6myc-rio1TEVpPGAL10-TEV Protease(red) andsir2Δcells (green) grown for eight divisions in 2% galactose medium. The rDNA array and ERCs are indicated. Right: quantified hybridization signals. (d) Fluorescence microscopy image of6myc-rio1TEVpPGAL10(left) and6myc-rio1TEVpPGAL10-TEV Protease(right) cells expressing Rad52-GFP and mCherry-Nop1. Scale bar, 5 μm. (e) Western blots of DNA checkpoint kinase Rad53 (anti-Rad53; anti-Pgk1=loading control) in6myc-rio1TEVpPGAL10(blue) and6myc-rio1TEVpPGAL10-TEV Protease(red) cells released from G1 in 2% galactose medium. (f) Western blots of Rad53 (anti-Rad53, anti-Pgk1=loading control) in6myc-rio1TEVpPGAL10(blue) and6myc-rio1TEVpPGAL10-TEV Protease(red) cells released from G1 in 2% galactose medium containing hydroxyurea. (g) Intranuclear distribution of Sir2 and condensin (subunit Smc2–3HA) as determined by IF imaging of spread nuclei (anti-Sir2 and anti-HA, respectively) isolated from of6myc-rio1TEVpPGAL10and6myc-rio1TEVpPGAL10-TEV Proteasecells released from G1 into the cell cycle (2% galactose medium).n=50 Per analysis. Figure 5: Rio1 promotes timely cell cycle commencement and rDNA stability. ( a ) 6myc-rio1 TEV p P GAL10 (blue) and 6myc-rio1 TEV p P GAL10 -TEV Protease (red) cells were arrested in G1 (2% raffinose). P GAL10 was then induced (1 h, 2% galactose) and the cells released into the cell cycle (2% galactose medium). Cells were tracked by analysis of spindle morphology (anti-Tub1 IF; n =200 cells per time point) and DNA content (FACS). The orange arrows indicate S phase. ( b ) Percentage of 6myc-rio1 TEV p P GAL10 (blue) and 6myc-rio1 TEV p P GAL10 -TEV Protease (red) cells, released from G1, with fragmented nucleoli (Nop1=nucleolar marker), as established by IF imaging analysis of spread nuclei (anti-myc, anti-Nop1). n =50 Per time point. Representative IF images are shown on the right. Scale bar, 5 μm. ( c ) Left: Southern blot (anti- 25S ) of total DNA isolated from 6myc-rio1 TEV p P GAL10 (blue), 6myc-rio1 TEV p P GAL10 -TEV Protease (red) and sir2Δ cells (green) grown for eight divisions in 2% galactose medium. The rDNA array and ERCs are indicated. Right: quantified hybridization signals. ( d ) Fluorescence microscopy image of 6myc-rio1 TEV p P GAL10 (left) and 6myc-rio1 TEV p P GAL10 -TEV Protease (right) cells expressing Rad52-GFP and mCherry-Nop1. Scale bar, 5 μm. ( e ) Western blots of DNA checkpoint kinase Rad53 (anti-Rad53; anti-Pgk1=loading control) in 6myc-rio1 TEV p P GAL10 (blue) and 6myc-rio1 TEV p P GAL10 -TEV Protease (red) cells released from G1 in 2% galactose medium. ( f ) Western blots of Rad53 (anti-Rad53, anti-Pgk1=loading control) in 6myc-rio1 TEV p P GAL10 (blue) and 6myc-rio1 TEV p P GAL10 -TEV Protease (red) cells released from G1 in 2% galactose medium containing hydroxyurea. ( g ) Intranuclear distribution of Sir2 and condensin (subunit Smc2–3HA) as determined by IF imaging of spread nuclei (anti-Sir2 and anti-HA, respectively) isolated from of 6myc-rio1 TEV p P GAL10 and 6myc-rio1 TEV p P GAL10 -TEV Protease cells released from G1 into the cell cycle (2% galactose medium). n =50 Per analysis. Full size image Through IF microscopy analysis of isolated nuclei, we next probed which rDNA regulators required nuclear Rio1 activity for their localization through the cell cycle. In short, cells lacking nuclear Rio1 had reduced levels of Sir2 at rDNA in interphase and metaphase, and of condensin in anaphase. The inability of these proteins to localize to the nucleolus led to their diffusion throughout the nucleus ( Fig. 5g , and Supplementary Figs 7 and 8 ). Reduced Sir2-mediated silencing of rDNA transcription [36] , [37] , required for sister rDNA alignment, may explain the observed rDNA-instability and array-expansion phenotype in yeast lacking nuclear Rio1 activity. As for condensin, this complex becomes highly enriched at anaphase rDNA to compact the array. Indeed, the large rDNA locus must be condensed before chromosome XII can move through the bud neck into the daughter cell [2] . In addition, condensin recruits topoisomerase II that resolves the remnant catenates lingering between the sister rDNA loci [2] , [3] , [4] , [7] . Both condensin-driven activities promote rDNA segregation in late anaphase. Indeed, live-cell microscopy revealed that yeast depleted of nuclear Rio1 was severely affected in its ability to segregate its GFP-marked rDNA loci ( Fig. 6a ). In contrast, centromere segregation was not affected ( Supplementary Fig. 9a ). Noteworthy, in cells lacking nuclear Rio1, the anaphase spindle (identified by mCherry-Tub1) extended till 11 μm (versus 7 μm in the control strain; Fig. 6a ), likely to try and segregate the rDNA loci. This phenotype is consistent with a defect in rDNA condensation [3] . 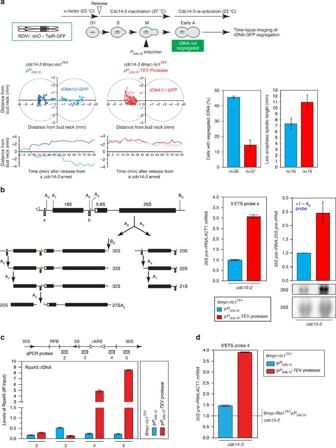Figure 6: Rio1 promotes rDNA segregation by downregulating RNA PolI. (a) The6myc-rio1TEVpPGAL10and6myc-rio1TEVpPGAL10-TEV Proteasestrains, carrying thecdc14-3allele and marked with a 256xtetO∼TetR-GFP array flankingRDN1(rDNA-GFP) were arrested in G1 (2% raffinose medium, 23 °C). Cells were then released into the cell cycle (2% raffinose medium, 37 °C) and arrested in early anaphase by inactivation of Cdc14-3. 2% Galactose was then added to inducePGAL10while the Cdc14-3 protein was re-activated in parallel (downshift to 23 °C). rDNA-GFP movement and segregation of the sister rDNA loci was tracked through anaphase by live-cell fluorescence microscopy. Left plots: single-cell rDNA segregation profiles. Projected movements of the sister rDNA arrays are shown in dark and light blue or in dark and light red colours. Right plots: percentage of cells with segregated sister rDNA-GFP loci, and the maximum length of their late-anaphase spindles. Error bars, s.d.’s.n=Indicated. (b) Sketch of 35S pre-RNA processing into 20S and 27SA2pre-rRNA. The graphs show the quantification of primary 35S rRNA levels measured by RT–qPCR (5′ETS probe 4) or by northern blot analysis (+1-A0probe) of cDNA or total RNA, respectively.6myc-rio1TEVcdc15-2cells carrying pPGAL10(blue) or pPGAL10-TEV Protease(red) were released from a metaphase arrest (nocodazole) underPGAL10-inducing conditions (37 °C). Error bars, s.d.’s.n=2. The northern blot with the +1-A0probe is shown underneath the graph. (c) ChIP–qPCR based measurement of Rpa43 levels at the rDNA ofcdc15-2 6myc-rio1TEVpPGAL10(blue) andcdc15-2 6myc-rio1TEVpPGAL10-TEV Proteasecells (red) arrested in anaphase following release from a metaphase arrest (37 °C, 2% galactose medium). Rpa43 levels across the rDNA unit were measured with probes 2–5. (d) RT–qPCR based quantification of primary 35S rRNA levels (5′ETS probe 4) in6myc-rio1TEVcdc14-3carrying pPGAL10(blue) or pPGAL10-TEV Protease(red) arrested in anaphase (37 °C) after release from a metaphase arrest (nocodazole) underPGAL10-inducing conditions. Reported values are normalized to the 35S levels measured forcdc15-2 6myc-rio1TEVpPGAL10cells, as indicated with a dashed line (Fig. 6b). Error bars, s.d.’s.n=3. Figure 6: Rio1 promotes rDNA segregation by downregulating RNA PolI. ( a ) The 6myc-rio1 TEV p P GAL10 and 6myc-rio1 TEV p P GAL10 -TEV Protease strains, carrying the cdc14-3 allele and marked with a 256x tetO ∼ TetR-GFP array flanking RDN1 (rDNA-GFP) were arrested in G1 (2% raffinose medium, 23 °C). Cells were then released into the cell cycle (2% raffinose medium, 37 °C) and arrested in early anaphase by inactivation of Cdc14-3. 2% Galactose was then added to induce P GAL10 while the Cdc14-3 protein was re-activated in parallel (downshift to 23 °C). rDNA-GFP movement and segregation of the sister rDNA loci was tracked through anaphase by live-cell fluorescence microscopy. Left plots: single-cell rDNA segregation profiles. Projected movements of the sister rDNA arrays are shown in dark and light blue or in dark and light red colours. Right plots: percentage of cells with segregated sister rDNA-GFP loci, and the maximum length of their late-anaphase spindles. Error bars, s.d.’s. n =Indicated. ( b ) Sketch of 35S pre-RNA processing into 20S and 27SA 2 pre-rRNA. The graphs show the quantification of primary 35S rRNA levels measured by RT–qPCR (5′ETS probe 4) or by northern blot analysis (+1-A 0 probe) of cDNA or total RNA, respectively. 6myc-rio1 TEV cdc15-2 cells carrying p P GAL10 (blue) or p P GAL10 -TEV Protease (red) were released from a metaphase arrest (nocodazole) under P GAL10 -inducing conditions (37 °C). Error bars, s.d.’s. n =2. The northern blot with the +1-A 0 probe is shown underneath the graph. ( c ) ChIP–qPCR based measurement of Rpa43 levels at the rDNA of cdc15-2 6myc-rio1 TEV p P GAL10 (blue) and cdc15-2 6myc-rio1 TEV p P GAL10 -TEV Protease cells (red) arrested in anaphase following release from a metaphase arrest (37 °C, 2% galactose medium). Rpa43 levels across the rDNA unit were measured with probes 2–5. ( d ) RT–qPCR based quantification of primary 35S rRNA levels (5′ETS probe 4) in 6myc-rio1 TEV cdc14-3 carrying p P GAL10 (blue) or p P GAL10 -TEV Protease (red) arrested in anaphase (37 °C) after release from a metaphase arrest (nocodazole) under P GAL10 -inducing conditions. Reported values are normalized to the 35S levels measured for cdc15-2 6myc-rio1 TEV pP GAL10 cells, as indicated with a dashed line ( Fig. 6b ). Error bars, s.d.’s. n =3. Full size image Rio1 downregulates PolI and stimulates pre-rRNA processing For rDNA to condensate and segregate, yeast must turn down PolI activity and locally resolve its transcripts before condensin can be loaded [1] , [4] . The Cdc14 phosphatase was previously shown to downregulate PolI in anaphase [4] . We wondered whether also Rio1 reduces PolI activity since our ChIP–qPCR analyses had identified high levels of 6myc-Rio1 at the 35S promoter and gene sequence in anaphase cells ( cdc15-2 ) (probes 4 and 5; Fig. 1e ). As such, we arrested the 6myc-Rio1 TEV cells in anaphase ( cdc15-2 ) following depletion of nuclear Rio1 activity at the metaphase–anaphase transition. RT–qPCR analysis of cDNA with a 5′-external transcribed spacer (5′ETS) probe (probe 4 in Fig. 6b ) revealed a threefold increase in 35S rRNA levels, as compared with the control anaphase cells. This result was confirmed by northern blot hybridization with a +1-A 0 probe showing a 2.5-fold increase in 35S rRNA concentrations ( Fig. 6b ), suggesting that Rio1 downregulates PolI activity in anaphase. To corroborate this conclusion, we localized PolI by ChIP–qPCR analysis of its subunit Rpa43 in anaphase-arrested cdc15-2 cells (37 °C) lacking or containing nuclear Rio1 activity. In the anaphase control cells, Rpa43 levels at the 35S promoter and gene sequence were low but increased by five- and eightfold, respectively, in the absence of nuclear Rio1 activity (red bars, Fig. 6c ). Combined, our PolI transcription and localization data indicate that Rio1 downregulates PolI activity in anaphase. The Cdc14 phosphatase reduces PolI activity by dissociating PolI from the anaphase rDNA [4] . Our Rpa43 ChIP data show an accumulation of PolI at the 35S unit in the absence of nuclear Rio1 activity, suggesting that Rio1 represses PolI transcription in a similar fashion. Since both the Cdc14 phosphatase [4] and Rio1 kinase downregulate PolI in anaphase, we next probed their relative contributions to this process. Whereas anaphase-arrested cells lacking Rio1 activity were characterized by a threefold increase in 35S rRNA concentrations ( Fig. 5b , probe 4), anaphase cells lacking Cdc14 activity ( cdc14-3 ) harboured only a 1.5-fold increase in 35S transcript levels as compared with cdc15-2 control cells ( Fig. 6d ), confirming previous findings [4] . Removing both Cdc14 and Rio1 activities led to a fourfold increase, indicating that both enzymes repress in parallel PolI transcription in anaphase. As Rio1 localizes to rDNA also before anaphase ( Fig. 1c–e ) and as PolI transcribes rDNA from G1 through metaphase [4] , we wondered whether Rio1 also modulates PolI transcription before anaphase. To answer this question, we arrested 6myc- rio1 TEV p P GAL10 - TEV Protease and 6myc- rio1 TEV p P GAL10 control cells in G1, depleted the cells of nuclear Rio1 activity and synchronously released them into the cell cycle. Variations in 35S transcript levels measured with the 5′ETS RT–qPCR probe were rather small in the control cells (low in S phase, slight increase in metaphase and slight decrease in anaphase; Fig. 7a and Supplementary Fig. 9b ). In contrast, marked changes were observed in the cells depleted of nuclear Rio1. Primary transcript levels were sevenfold elevated in G1, then decreased through S phase (still 3.5-fold above the levels measured in the S phase control cells) and increased threefold in anaphase. This transcript–concentration profile is consistent with Rio1 localizing to the rDNA ( Fig. 1c–e ) to reduce PolI activity through the cell cycle. 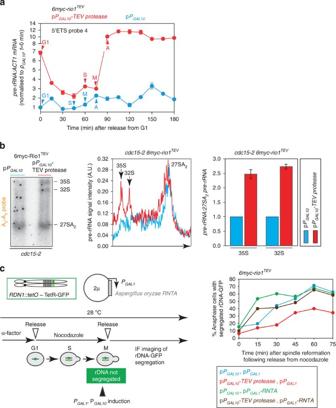Figure 7: Rio1 promotes rDNA segregation by removing RNA PolI and by stimulating the nucleolar processing of pre-rRNA transcripts. (a) RT–qPCR analysis of 35S cDNA (5′ETS probe 4) from6myc-rio1TEVpPGAL10(blue) and6myc-rio1TEVpPGAL10-TEV Protease(red) cells synchronously released from G1 into the cell cycle (2% galactose medium).PGAL10was induced 1 h before releasing the G1 arrested cells. Error bars, s.d.’s.n=3. (b) Left: northern blot analysis with an A2-A3probe of total RNA isolated from6myc-rio1TEVcdc14-3cells carrying pPGAL10(blue) or pPGAL10-TEV Protease(red). The cells were arrested in anaphase after release from a metaphase arrest (nocodazole, 23 °C) underPGAL10-inducing conditions (37 °C). Right: quantified northern blot signals, and 35S and 32S pre-rRNA levels relative to those of 27SA2pre-rRNA. (c)6myc-rio1TEVpPGAL10and6myc-rio1TEVpPGAL10-TEV Proteasecells marked with a 256xtetO∼TetR-GFP array atRDN1, containing the pPGAL1-A. oryzae RNTAor the pPGAL1control vector. The strains were arrested in metaphase (nocodazole) and released into anaphase underPGAL1- andPGAL10-inducing conditions (2% galactose medium). rDNA-GFP segregation was tracked through anaphase by live-cell fluorescence microscopy (n=30 cells per time point). Figure 7: Rio1 promotes rDNA segregation by removing RNA PolI and by stimulating the nucleolar processing of pre-rRNA transcripts. ( a ) RT–qPCR analysis of 35S cDNA (5′ETS probe 4) from 6myc-rio1 TEV p P GAL10 (blue) and 6myc-rio1 TEV p P GAL10 -TEV Protease (red) cells synchronously released from G1 into the cell cycle (2% galactose medium). P GAL10 was induced 1 h before releasing the G1 arrested cells. Error bars, s.d.’s. n =3. ( b ) Left: northern blot analysis with an A 2 -A 3 probe of total RNA isolated from 6myc-rio1 TEV cdc14-3 cells carrying p P GAL10 (blue) or p P GAL10 -TEV Protease (red). The cells were arrested in anaphase after release from a metaphase arrest (nocodazole, 23 °C) under P GAL10 -inducing conditions (37 °C). Right: quantified northern blot signals, and 35S and 32S pre-rRNA levels relative to those of 27SA 2 pre-rRNA. ( c ) 6myc-rio1 TEV p P GAL10 and 6myc-rio1 TEV p P GAL10 -TEV Protease cells marked with a 256x tetO ∼ TetR-GFP array at RDN1 , containing the p P GAL1 - A. oryzae RNTA or the p P GAL1 control vector. The strains were arrested in metaphase (nocodazole) and released into anaphase under P GAL1 - and P GAL10 -inducing conditions (2% galactose medium). rDNA-GFP segregation was tracked through anaphase by live-cell fluorescence microscopy ( n =30 cells per time point). Full size image To ensure rDNA segregation, yeast must not only reduce PolI activity but also locally resolve the PolI-generated transcripts. During our earlier northern blot analysis of 20S pre-rRNA processing in exponential cells depleted for 3 h of nuclear Rio1 activity (D-A 2 probe in Fig. 4e ), we had noticed that the cells accumulated 32S rRNA transcripts ( Supplementary Fig. 9d ), indicating a defect in 32S cleavage at A 2 by the nucleolar SSU processome and associated factors [5] , [38] , [39] , [40] . As such, we probed rRNA transcript processing in our anaphase-arrested cells ( cdc15-2) depleted of Rio1 activity. Northern hybridization of total rRNA with an A 2 -A 3 probe revealed a 2.5-fold increase in 35S and 32S pre-RNA levels ( Fig. 7b ), indicating a derepressed PolI activity and a defect in nascent transcript processing at A 2 . To determine whether the accumulation of pre-rRNA impaired rDNA segregation in yeast depleted of nuclear Rio1, we tracked rDNA-GFP through anaphase in 6myc-rio1 TEV p P GAL10 and 6myc-rio1 TEV p P GAL10 -TEV Protease cells that inducibly expressed the Aspergillus oryzae ribonuclease RntA [4] , [41] from P GAL1 ( Fig. 7c ). We observed that the RntA-mediated degradation of the accumulated rRNA transcripts ( Supplementary Fig. 9e ) promoted rDNA segregation in yeast depleted of nuclear Rio1 ( Fig. 7c ). As such, rDNA transmission occurs only when Rio1, together with Cdc14, downregulates PolI activity and then stimulates the co-transcriptional processing of nascent transcripts in the nucleolus. Rio1 reduces PolI activity by targeting subunit Rpa43 Transcription factor Rrn3 recruits PolI to the 35S promoter via PolI subunit Rpa43, an event that converts inactive PolI into an initiation-competent PolI (ref 42 , 43 ). In anaphase, the Cdc14 phosphatase downregulates PolI by dephosphorylating Rpa43, resulting in PolI dissociating from the anaphase rDNA [4] . To examine whether Rio1 also dislodges PolI by targeting Rpa43, we first probed their physical interaction and found that 6myc-Rio1 and Rpa43-3HA efficiently co-immunoprecipitated from exponentially growing cells ( Fig. 8a ). Next, PhosTag western blot analysis of Rpa43-3HA in 6myc-rio1 TEV p P GAL10 -TEV Protease and 6myc - rio1 TEV p P GAL10 cells identified a slow-migrating, anaphase-specific Rpa43-3HA phospho species that was absent in the cells lacking nuclear Rio1 activity ( Fig. 8b ). To further associate this anaphase-specific Rpa43 phospho species with Rio1 kinase activity, we analysed Rpa43 phosphorylation in cells expressing either a dominant-negative kinase-dead rio1 allele ( P GAL1 - rio1 D244A ) or wild-type RIO1 ( P GAL1 - RIO1 ) (ref. 12 ). PhosTag western blot analysis showed that the cells expressing rio1 D244A lacked the slow-migrating Rpa43-3HA phospho species in anaphase ( Fig. 8c ). To examine whether Rio1 directly phosphorylates Rpa43, we performed an in vitro kinase assay with recombinant His6-Rio1 and Rpa43-His6-HA purified from Escherichia coli ( Supplementary Fig. 9f ) and found that Rpa43 was phosphorylated only in the presence of Rio1 ( Fig. 8d ). Interestingly, Rio1 autophosphorylation [12] , [22] was threefold (3.1±0.6) higher in the presence of Rpa43, indicating that Rio1 binding to Rpa43 may have stimulated its own phosphorylation, which in turn may have promoted the phosphorylation of Rpa43 (the protein loading controls for the kinase assay are shown in Supplementary Fig. 9g ). Finally, we sought to identify the Rpa43 residues targeted by Rio1 using mass spectrometry. After repeating the in vitro kinase assay in the presence and absence of unlabelled ATP, nanoLC-MS/MS analysis [44] (98.8% combined peptide coverage) found Rpa43 phospho-peptide QHLNPLVMK Y73 NNK to be threefold (3.2±0.3) enriched over the negative-control peptide (unphosphorylated peptides were 1.1- to 1.3-fold upregulated versus their counterparts in the negative-control Rpa43 species; Fig. 8e ). Tyrosine 73 was the sole Rpa43 residue found to be phosphorylated. Although no physiological substrates of Rio1 have yet been identified, Rio1 kinases are considered serine kinases as Archeoglobus fulgidus Rio1 phosphorylates itself at S108 (ref. 45 ) and because S. cerevisiae Rio1 phosphorylates serines in casein and in itself (residues not identified) [21] . However, recent studies suggested that RIO kinases can perform autophosphorylation at aspartate [12] , [13] , within the RIO domain. Our findings further indicate that Rio1 phosphorylation activity is wide ranging and may harbour serine/tyrosine dual specificity, as observed for canonical kinases CK2 (refs 46 , 47 ), Hrr25 (ref. 48 ), Mps1 (ref. 49 ), Rad53 (ref. 50 ), Dusty [51] and Swe1 (ref. 52 ). Tyrosine 73 is one of the few evolutionary conserved residues present in Rpa43 ( Fig. 8f and Supplementary Fig. 10 ) and resides–from a regulatory point of view—at a highly strategic position. Indeed, within Rpa43, Y73 lies in a short N-terminal β-strand proximal to six C-terminal β-strands and one α-helix that are enriched with phosphorylated residues, as identified by mass spectrometric analysis of Rpa43 isolated from yeast [53] , [54] , [55] . Y73 flanks K72 and lies near G78 and L87G88Y89, putative interaction points that may mediate Rpa43-Rpa14 heterodimer formation within PolI (refs 56 , 57 ). In addition, Y73 lies in close proximity to the negatively charged residues emanating from the C-terminus of Rpa135 ( Fig. 5g ). As such, Rio1 kinase activity could induce a charge-based repulsion and destablization of protein interactions within the polymerase complex. The N-terminal domain of Rpa43 that harbours Y73 also binds to the PolI-recruiting transcription factor Rrn3 (ref. 53 ). Taken together, our cell biological and biochemical data indicate that Rio1 phosphorylates Rpa43 in anaphase to remove PolI from the rDNA. Whether this clearance occurs via disruption of the Rpa43—Rrn3 interaction or via the dissolution of intra-PolI contacts will be determined in future research. 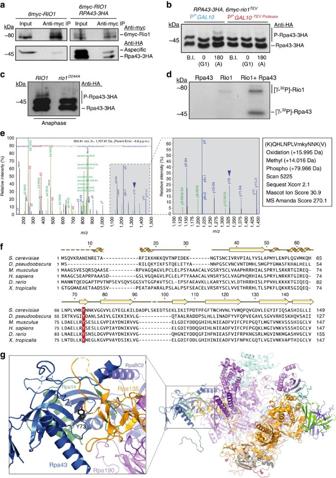Figure 8: Rio1 downregulates RNA PolI by targeting subunit Rpa43. (a) 6myc-Rio1 and Rpa43-3HA co-immunoprecipitate from whole-cell extract derived from exponentially growing6myc-RIO1RPA43-3HAcells. (b) PhosTag western blot of Rpa43-3HA (anti-HA) in6myc-rio1TEVpPGAL10(blue) and6myc-rio1TEVpPGAL10-TEV Protease(red) cells. Cells were collected beforePGAL10induction (B.I.), after 1 h of induction during the G1 arrest (G1), and 3 h after the release from G1 (anaphase, A). (c) PhosTag western blot of Rpa43-3HA (anti-HA) inRPA43-3HAcells inducibly expressing wild-typeRIO1or the dominant-negative kinase-deadrio1D244Aallele fromPGAL1on a 2 μ plasmid. The cells were collected in anaphase 3 h after release from G1 in 2% galactose medium. (d)In vitrokinase assay with recombinant His6-Rio1 (1 μg) and recombinant Rpa43-His6-HA (6 μg) in the presence of 0.05 μM [γ-32P]ATP. The radiographs show phosphorylated His6-Rio1 and Rpa43-His6-HA. (e) NanoLC-MS/MS spectrum of the Rpa43 QHLNPVMKY73NNK phospho-peptide. The position of phospho-Y73 is indicated with an arrowhead. (f) Alignment of the Rpa43 proteins fromSaccharomyces cerevisiae,Drosophila pseudoobscura,Mus musculus,Homo sapiens,Dario rerioandXenopus tropicalis(UniProtKB database entries: A6ZPH0, Q29JY4, Q78WZ7, Q3B726, Q6PHG8 and F7BDD1, respectively) using Muscle (www.ebi.ac.uk/Tools/msa/muscle). TheS. cerevisiaeY73 residue and its equivalents in the Rpa43 orthologues are indicated in white font on a red background. (g) Localization of Rpa43 Y73, indicated in black, within the 14-subunit RNA PolI enzyme complex57(top view rotated +90°; PDB 4C3J). Figure 8: Rio1 downregulates RNA PolI by targeting subunit Rpa43. ( a ) 6myc-Rio1 and Rpa43-3HA co-immunoprecipitate from whole-cell extract derived from exponentially growing 6myc-RIO1 RPA43-3HA cells. ( b ) PhosTag western blot of Rpa43-3HA (anti-HA) in 6myc-rio1 TEV p P GAL10 (blue) and 6myc-rio1 TEV p P GAL10 -TEV Protease (red) cells. Cells were collected before P GAL10 induction (B.I. ), after 1 h of induction during the G1 arrest (G1), and 3 h after the release from G1 (anaphase, A). ( c ) PhosTag western blot of Rpa43-3HA (anti-HA) in RPA43-3HA cells inducibly expressing wild-type RIO1 or the dominant-negative kinase-dead rio1 D244A allele from P GAL1 on a 2 μ plasmid. The cells were collected in anaphase 3 h after release from G1 in 2% galactose medium. ( d ) In vitro kinase assay with recombinant His6-Rio1 (1 μg) and recombinant Rpa43-His6-HA (6 μg) in the presence of 0.05 μM [γ- 32 P]ATP. The radiographs show phosphorylated His6-Rio1 and Rpa43-His6-HA. ( e ) NanoLC-MS/MS spectrum of the Rpa43 QHLNPVMKY73NNK phospho-peptide. The position of phospho-Y73 is indicated with an arrowhead. ( f ) Alignment of the Rpa43 proteins from Saccharomyces cerevisiae , Drosophila pseudoobscura , Mus musculus , Homo sapiens , Dario rerio and Xenopus tropicalis (UniProtKB database entries: A6ZPH0, Q29JY4, Q78WZ7, Q3B726, Q6PHG8 and F7BDD1, respectively) using Muscle ( www.ebi.ac.uk/Tools/msa/muscle ). The S. cerevisiae Y73 residue and its equivalents in the Rpa43 orthologues are indicated in white font on a red background. ( g ) Localization of Rpa43 Y73, indicated in black, within the 14-subunit RNA PolI enzyme complex [57] (top view rotated +90°; PDB 4C3J). Full size image We have identified Rio1 as a cell cycle-driven regulator of rDNA transcription, pre-rRNA processing, rDNA stability and segregation ( Fig. 9 ). Yeast SSU processome mutants arrest at cell cycle entry (START) because pre-rRNA does not become processed and ribosomes are not being synthesized [58] . Our cell cycle experiments revealed that G1 cells lacking nuclear Rio1 activity accumulate primary 35S transcripts but also pre-rRNA species not yet processed at A 2 (RT–qPCR analysis with a probe covering the A 2 site; Supplementary Fig. 9c ). These anomalies may help to explain the delay at START of our mutant. 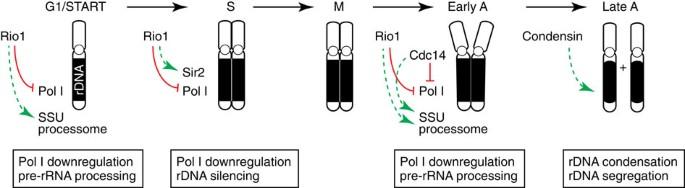Figure 9: Rio1 downregulates RNA PolI to promote rDNA stability and segregation. Working model of Rio1-mediated regulation of rDNA transcription, pre-rRNA processing, rDNA stability and segregation, as identified in this study. In G1, Rio1 downregulates 35S rDNA transcription by PolI and promotes pre-rRNA processing at A2by the SSU processome and associated factors, allowing for a timely commencement of the cell cycle at START. In S phase, the Rio1-mediated downregulation of PolI and recruitment of the histone deacetylase Sir2 to rDNA chromatin, promote rDNA stability. As rDNA replication progresses, Rio1 concentrations at S phase rDNA decrease, resulting in metaphase nuclei containing low levels of Rio1. At anaphase onset, Rio1 becomes re-recruited to the nucleolus to remove PolI from the rDNA by targeting PolI subunit Rpa43. PolI delocalization and promotion of pre-rRNA processing at the rDNA allow for condensin enrichment, resulting in rDNA compaction and segregation. Red lines: inhibitory activity, green lines: activating activity, solid lines: direct activity, dashed lines: direct or indirect activity. Figure 9: Rio1 downregulates RNA PolI to promote rDNA stability and segregation. Working model of Rio1-mediated regulation of rDNA transcription, pre-rRNA processing, rDNA stability and segregation, as identified in this study. In G1, Rio1 downregulates 35S rDNA transcription by PolI and promotes pre-rRNA processing at A 2 by the SSU processome and associated factors, allowing for a timely commencement of the cell cycle at START. In S phase, the Rio1-mediated downregulation of PolI and recruitment of the histone deacetylase Sir2 to rDNA chromatin, promote rDNA stability. As rDNA replication progresses, Rio1 concentrations at S phase rDNA decrease, resulting in metaphase nuclei containing low levels of Rio1. At anaphase onset, Rio1 becomes re-recruited to the nucleolus to remove PolI from the rDNA by targeting PolI subunit Rpa43. PolI delocalization and promotion of pre-rRNA processing at the rDNA allow for condensin enrichment, resulting in rDNA compaction and segregation. Red lines: inhibitory activity, green lines: activating activity, solid lines: direct activity, dashed lines: direct or indirect activity. Full size image In S phase, Rio1 acts at multiple levels. By tuning down transcription by PolI, Rio1 may reduce the frequency of collisions between the replisome and PolI within the 35S sequence, hence minimizing the production of double-strand breaks and incomplete transcripts [59] . Excessive PolI activity may also lead to extreme supercoiling and aberrant chromatin structures that stimulate DNA breakage and recombination. During rDNA replication, the RFB-bound proteins prevent the replisome from entering the 35S rDNA sequence and promote a correct alignment of the newly replicated sister rDNA arrays. Their recruitment of Rio1 indicates an involvement of the kinase in regulating these RFB activities. Rio1 also localizes the histone deacetylase Sir2 to rDNA chromatin. Sir2 promotes rDNA stability by localizing both to the RFB and also to the cryptic E-Pro promoter. By repressing PolII-mediated transcription from E-Pro, Sir2 prevents the synthesis of non-coding E-Pro transcripts that displace the cohesin complexes and cause the sister arrays to misalign [36] . Double-strand rDNA breaks repaired by recombination between misaligned sister arrays results in rDNA repeat-number expansion or reduction, and in the formation of ERCs [27] , [28] . Both ERC accumulation and rDNA repeat-number instability have been linked to senescence (shortened lifespan) [29] , [30] , suggesting that Rio1 may determine yeast life expectancy. When rDNA repeat numbers fall below wild-type level, reduced repression of E-Pro may promote unequal recombination and increase repeat numbers. As such, Rio1 could act as a monitor of rDNA copy number and as an array manager by dictating Sir2 levels and activity. Once cells have endured rDNA replication, repression of PolI activity may no longer be necessary in metaphase. As such, Rio1 dissociating from the metaphase nucleolus may lead to a temporal increase in rDNA transcription before PolI becomes downregulated in anaphase. Rio1, together with the conserved Cdc14 phosphatase, reduce PolI activity by targeting Rpa43, a subunit of the Rpa14-Rpa43 dimer, that lies at the outer edge of PolI and mediates PolI recruitment by Rrn3 (refs 42 , 43 ). The concurrent action by Rio1 and Cdc14 may establish a local phospho-threshold that commands the dissociation of PolI from 35S at anaphase entry. By downregulating PolI and by stimulating PolI transcript processing at the A 2 site (as mediated by the SSU processome), Rio1 promotes condensin binding and rDNA transmission. Indeed, without Rio1 activity, the long right arm of chromosome XII harbouring the rDNA array does not segregate into the daughter cells, resulting in chromosome loss. We also observed that condensin itself recruits Rio1 to anaphase rDNA, suggesting that Rio1 might also promote condensin activity. The monopolin complex, which tethers the nucleolus to the nuclear membrane via the CLIP (Chromosome Linkage Inner nuclear membrane Protein) complex [48] , also recruits Rio1 to anaphase rDNA. It is tempting to speculate that Rio1 targeting monopolin may facilitate rDNA segregation by inducing rDNA detachment from the nuclear envelope. Rio1 and its human orthologue RIOK1 promote the endonucleolytic cleavage of 20S pre-rRNA at pre-40S ribosomes, and stimulate the recycling of trans-acting factors that catalyse 40S maturation [12] , [18] , [19] , [20] . While these events occur in the cytoplasm, a small pool of RIOK1 also localizes to the human nucleus [19] , [20] . Treating murine cells with toyocamycin, an inhibitor of Rio1 activity in vitro [61] , impeded nucleolar pre-rRNA processing [62] , indicating that RIOK1 might be involved in early pre-rRNA cleavage, as we observed for Rio1 in yeast. In contrast to yeast, vertebrate cells contain five rDNA clusters on different chromosomes. In prophase, these nucleoli disassemble and their transcription becomes repressed to allow the stripped rDNA to segregate with the rest of the genome. Nucleolar transcription is downregulated by the CDK1-cyclin B kinase, whose phosphorylation of promoter selectivity factor SL1 prevents the formation of the PolI pre-initiation complex [63] , [64] , [65] . Similar to yeast Rio1, RIOK1 might just as well contribute to the transcriptional repression of PolI. In conclusion, our study reveals the first nuclear functions of the Rio1 kinase. By downregulating PolI-mediated rDNA transcription and by promoting the processing of its transcripts, Rio1 ensures both a timely commencement and conclusion of the cell cycle (rDNA segregation permits exit from mitosis). Rio1 safeguards rDNA stability during DNA replication and integrates early nucleolar and late cytoplasmic events during ribosome biogenesis. As such, Rio1 activity allows yeast to actively grow and divide while ensuring the integrity and faithful transmission of its genome. Yeast strains Yeast strains (W303-1A background; Supplementary Table 1 ) were made by mating, tetrad dissection and spore selection, by introducing integrative or episomal plasmids or via transformation and homologous recombination of PCR-generated deletion or epitope cassettes. None of the epitopes affected yeast fitness or the activity of the tagged protein. The plasmids used in this study are listed in Supplementary Table 2 . To generate the 6myc-rio1 TEV strain, 21 nucleotides (5′-GAAAACCTGTATTTTCAGGGC-3′) encoding the TEV Protease cleavage site (ENLYFQG) were introduced by PCR between the nucleotides encoding Rio1 residues E406 and E407 in an integrative URA3 -based plasmid harbouring 6myc-RIO1 under control of its endogenous promoter, P RIO1 . After linearization in P RIO1 by the endonuclease SgraI, the plasmid was integrated at the endogenous P RIO1 in the genome of parent strain PDW001. Following incubation on complete minimal medium containing 1 g l −1 5-fluoroorotic acid (Fluka), we PCR-identified the colonies in which wild-type RIO1 had been recombined out, leaving the 6myc-rio1 allele expressed from P RIO1 and harbouring the TEV Protease cleavage site (named 6myc-rio1 TEV ) as the only source of Rio1. The episomal high-copy 2 μ p P GAL10 -HA-TEV Protease-NLS plasmid was made by subcloning the HA-TEV Protease-NLS sequence from pYeF1-TEV (ref. 66 ) into the HIS3 -marked P GAL10 expression plasmid pYeHFc2H (p P GAL10 , gift from C. Cullin) as well as into pYeHFc2H provided with geneticin-resistance cassette KanMX4 . After transforming the 6myc-rio1 TEV strain, we obtained strain 6myc-rio1 TEV p P GAL10 -TEV Protease and the 6myc-rio1 TEV p P GAL10 control strains. Cell cycle studies Cells were grown at 23 °C in minimal synthetic drop-out media or in YEPA medium (1% yeast extract, 2% peptone and 0.3 mM adenine) containing 2% raffinose, 2% galactose or 2% glucose. To arrest yeast in G1, S phase or metaphase, cultures were treated (2.5–3 h) with 5 μg ml −1 α-factor (GeneScript), 10 μg ml −1 hydroxyurea (Sigma-Aldrich) or 15 μg ml −1 nocodazole (Sigma-Aldrich), respectively. To release the cells into the cell cycle, we filtered the yeast cultures, washed and then resuspended the cells in drug-free medium. To arrest the cells in anaphase, strains carrying either the temperature-sensitive cdc15-2 or cdc14-3 allele were first arrested in G1 or metaphase (23 °C) and then released at the non-permissive temperature (37 °C). To deplete Rio1 activity from the nucleus, both the 6myc-rio1 TEV p P GAL10 -TEV Protease strain and the 6myc-rio1 TEV p P GAL10 negative-control strain were grown in 2% raffinose YEPA medium (raffinose does not affect P GAL10 ) containing 220 μg ml −1 geneticin (G418, Life Technologies). While arrested or during exponential growth, the cells were treated with 2% galactose to induce P GAL10 (for 1 h during the arrest, for 3 h during exponential growth). Arrested cells were then released in medium containing 2% galactose, 2% raffinose and 220 μg ml −1 G418. For rDNA and ERC analysis, total DNA was extracted from cells grown for 15 h (eight divisions) in 2% galactose medium, run on a 0.6% TBE-agarose gel, transferred for Southern blot analysis and hybridized with a 25S rDNA probe [32] . The oligomers used to produce the probe are listed in Supplementary Table 3 . Progression through the cell cycle was tracked by indirect IF microscopy analysis of spindle morphology (see further down) and by FACS analysis of DNA content. Regarding the latter, cells were fixed in 70% ethanol, incubated first with 1 mg ml −1 RNAse A (Sigma-Aldrich), then with 5 mg ml −1 pepsin (Sigma-Aldrich) and ultimately resuspended in 1 mg ml −1 propidium iodide (Sigma-Aldrich). After mild sonication, cell fluorescence was analysed with a FACScan (Becton Dickinson) sorter and DNA content profiles generated with CellQuest software. IF imaging of yeast cells was performed with 1 ml of cell culture. The cells were centrifuged and crosslinked overnight in 1 ml of 3.7% formaldehyde. The cell walls were then digested (30 min) with zymolyase (100 μg ml −1 , Amsbio), washed with 1.2 M sorbitol and 100 mM phospho-citrate, pH 5.9, and bound to a multiwall poly- L -lysine-coated glass slide (Sigma-Aldrich). The slide was treated with DAPI and hybridized with rat monoclonal anti-Tub1 (YOL1/34, Adb Serotec MCA78G), rabbit polyclonal anti-GFP (Life Technologies,A-6455), goat polyclonal anti-Cdc14 (yE-17, Santa Cruz Biotech sc-12045) or mouse monoclonal anti-myc (9E10, Covance MMS-150R) primary antibodies. CY3 (715-165-151)- or fluorescein isothiocyanate (FITC; 111-095-144)-labelled secondary antibodies (Jackson Laboratory) were used to visualize the proteins. IF imaging of rDNA or centromeres in fixed cell samples was done as described above and performed with strains whose RDN1 or CEN4 sequence was flanked with a 256x tetO ∼ TetR-GFP array. Images were acquired with a DeltaVision ELITE microscope (Applied Precision) carrying an Olympus IX71 UPlanSApo objective lens (numerical aperture 1.40) and a CoolSnap HQ2 CCD Camera (Photometrics). Fifteen Z-stacks were acquired every 0.4 μm, deconvoluted (SoftWoRx) and projected with maximum intensity. IF imaging of spread nuclei was performed using 4 ml of cell culture. The cells were centrifuged and digested with zymolyase (30 μg ml −1 ). The spheroblasts were then fixated on a glass slide with 4% paraformaldehyde and 3.4% sucrose, and spread with a glass rod. The slides were then hybridized with rabbit polyclonal anti-GFP (Life Technologies A-6455), mouse monoclonal anti-HA (16B12, Covance MMS-101P), mouse monoclonal anti-myc (9E10, Covance MMS-150R), mouse monoclonal anti-Nop1 (28F2, EnCore Biotech MCA28F2), rabbit polyclonal anti-Rio1 (gift from J.-P. Gelugne) or goat polyclonal anti-Sir2 (yN-19, Santa Cruz Biotech sc-6666) antibodies. CY3- or FITC-labelled secondary antibodies (Jackson Laboratory, see above) were used. Nuclei were imaged with a BX51 wide-field fluorescence microscope (Olympus). Live-cell imaging of spindle (mCherry-Tub1) elongation and RDN1 -GFP segregation was performed with microfluidic plates (CellASIC) and a DeltaVision microscope setup as described above via 15 Z-stacks (0.4 μm each). The images were deconvoluted (SoftWoRx), projected with maximum intensity and analysed with ImageJ1.43u (National Institutes of Health, N.I.H.). Immunobloting Cells were collected, treated with 5% trichloroacetic acid (TCA), resuspended in lysis buffer (50 mM Tris-Cl pH7.5, 1 mM EDTA.Na 2 , 50 mM dithiothreitol, 60 mM β-glycerophosphate, 0.1 mM Na 3 VO 4 and 5 mM NaF) containing protease inhibitors (Roche) and then disrupted with glass beads and a FastPrep-24 instrument (MP Biomedicals). Lysates were cleared by centrifugation, resuspended in sample loading buffer (8% SDS, 200 mM Tris-Cl, pH 6.8, 400 mM dithiothreitol, 0.4% bromophenol blue and 40% glycerol), heat-denatured and run on SDS polyacrylamide gels. To separate the phospho species of Rpa43-3HA, the SDS polyacrylamide gels were provided with 30 μM PhosTag (Manac Incorporated). Proteins were transferred onto Immobilon-P membranes (Millipore) and incubated with mouse monoclonal anti-Pgk1 antibody (1:5,000; Life Technologies 459250), mouse monoclonal anti-Rad53 EL7E1 (4 μg ml −1 , gift from M. Foiani), goat polyclonal anti-Cdc14 yE-17 (1:1,000; Santa Cruz sc-12045), mouse monoclonal anti-Flag M2 (1:4,000; Sigma-Aldrich A2220), mouse monoclonal anti-Myc 9E10 (1:1,000; Covance MMS-150R), mouse monoclonal anti-HA 16B12 (1:1,000; Covance MMS-101P) or mouse monoclonal anti-HIS H-3 (1:200, Santa Cruz sc-8036) antibodies. Horseradish peroxidase (HRP)-conjugated goat anti-mouse (1:10,000; Bio-Rad 170–6516) or goat anti-rabbit (1:10,000; Bio-Rad 170–6515) secondary antibodies were used to visualize the proteins with ECL chemiluminescence (GE Healthcare) and radiography film (GE Healthcare). Uncropped blots are shown in Supplementary Fig. 11 . To probe the interaction between 6myc-Rio1 and Rpa43-3HA or between 6myc-Rio1 and Sgs1-3FLAG, yeast whole-cell extract (3 μg of total protein) was incubated with anti-myc sepharose matrix (9E10, Covance AFC-150P) or anti-HA sepharose matrix (3F10, Roche 11815016001). Following four washes with high salt and detergent buffer (50 mM HEPES, pH 7.5, 500 mM NaCl, 2.5 mM MgCl 2 , 0.5% Nonidet P (NP)-40 and 10% glycerol), Rpa43-3HA, 6myc-Rio1 or Sgs1-3Flag were visualized by western hybridization analysis. Rio1 kinase activity measurements To measure the kinase activity of full-length or truncated 6myc-Rio1 TEV , cells were grown in 2% raffinose medium, arrested in G1 and collected before, upon and after P GAL10 induction with 2% galactose. Cells were resuspended in lysis buffer (50 mM HEPES-KOH, pH 7.1, 50% glycerol, 300 mM NaCl, 1% NP-40, 1 mM Na3VO4, 1 mM NaF and 1 mM phenylmethylsulfonyl fluoride (PMSF)) and whole-cell extracts made with glass beads. Cleared extract (500 μg of protein) was then incubated (4 °C, overnight) with anti-myc sepharose beads (Covance). The beads were washed once with washing buffer (50 mM HEPES-KOH, pH 7.1, 300 mM NaCl, 1% NP-40, 1 mM Na 3 VO 4 , 1 mM NaF and 1 mM PMSF), and three times with kinase buffer (50 mM HEPES-KOH, pH 7.2, 5 mM MgCl 2 and 5 mM MnCl 2 ). Bead-bound 6myc-Rio1 TEV was incubated with 1.5 mg ml −1 of dephosphorylated casein (Sigma-Aldrich) and 0.03 μM [γ-32P]ATP (PerkinElmer) in kinase buffer. The assay (15 min, 24 °C) was performed in the presence or absence of CK1 and CK2 kinase inhibitors (5 μM each; CKI-7 dichlorhydrate and 4,5,6,7-tetrabromobenzotriazole (TBB), respectively; Sigma-Aldrich). The reactions were analysed on SDS polyacrylamide gels, which were then fixed in a 30% methanol+10% acetic acid solution, and dried on a Gel Dryer (Bio-Rad). The phospholabelled proteins were visualized by autoradiography and quantified using ImageJ. RT–qPCR analysis of rRNA Total RNA was isolated [67] from cells collected through the cell cycle or enriched at a specific cell cycle stage. RNA (1 μg) was retrotranscribed into cDNA with Random Primers (Life Technologies) and ImProm-II Reverse Transcriptase (Promega). cDNA (5 ng) was analysed by RT–qPCR analysis (7500 Fast Real-Time PCR, Life Technologies) using TaqMan probes (Life Technologies; Supplementary Table 3 ) against the 5′ETS sequence of 35S pre-rRNA (probe 4 in the figures) or against the A 2 -processing site of 35S, 33S and 32S pre-rRNA (probe 6). ACT1 cDNA (housekeeping control) was used as the internal reference. Analyses were done in triplicate. ChIP–qPCR analysis For each analysis, 50 ml of cell culture were treated with 1% formaldehyde (2 h). Crosslinked cells were washed with Tris-buffered saline (50 mM Tris-Cl, pH 7.5, 150 mM NaCl) and resuspended in lysis buffer (50 mM HEPES, pH 7.5, 140 mM NaCl, 1 mM EDTA, 1% Triton X-100 and 0.1% sodium deoxycholate). The cells were broken with glass beads and the whole-cell extracts were sonicated on ice with a Branson Sonifier 250 (5 × 30 s, 2 min on ice) to reduce the genome in ∼ 500 bp fragments. Anti-myc sepharose beads and rabbit polyclonal anti-Rpa43 antibody (gift from M. Riva) conjugated to protein A-associated agarose beads (Pierce) were incubated (4 °C, overnight) with the extracts to isolate 6myc-Rio1 and Rpa43. The beads were then washed twice with lysis buffer, once with washing buffer (100 mM Tris-Cl, pH 8.0, 1 mM EDTA 1% Triton X-100, 0.1% sodium deoxycholate, 0.5% NP-40 and 250 mM LiCl) and once with TE buffer. The beads were resuspended (10 min, 65 °C) in elution buffer (1% SDS, 50 mM Tris-Cl, pH 8.0, 10 mM EDTA) and the eluted material then separated from the beads and heated (65 °C, overnight) to reverse the crosslinks. An amount of 25 μl of total chromatin solution were similarly heat treated (=Input). After treatment with 20 mg ml −1 proteinase K (Roche), the material was treated with 10 mg ml −1 RNase (Sigma-Aldrich) for 30 min at 37 °C, and the DNA was extracted with phenol and chloroform. Following precipitation, the DNA was resuspended in 40 μl water. Input and immunoprecipitated samples were analysed by RT–qPCR (probes are indicated in the Figures 1a, 6b and 6c and in Supplementary Table 3 ). Yeast two-hybrid interaction screens Yeast two-hybrid screens were performed by Hybrigenics Services ( www.hybrigenics-services.com ). The RIO1 coding sequence (YOR119C) was cloned as a C-terminal fusion to LEXA or the GAL4 encoding DNA-binding domain, or as an N-terminal fusion to LEXA or GAL4 . The constructs were screened by mating and covered the complexity of the S. cerevisiae genomic library 5- to 14-fold. Prey fragments of positive clones were amplified by PCR, sequenced and the interacting sequences were identified in the GenBank database (NCBI). Ribosome, protein translation and northern blot analysis For ribosome profiling, 6myc-rio1 TEV p P GAL10 and 6myc-rio1 TEV p P GAL10 -TEV Protease cells were grown exponentially in 2% raffinose medium to an OD 600 =0.5. Galactose (2%) was added and samples were taken at the indicated time points and treated on ice (5 min) with 100 μg ml −1 cycloheximide to stabilize the polysomes. The cells were washed with extraction buffer (20 mM Tris-Cl, pH 7.5, 50 mM KCl, 10 mM MgCl 2 and 100 μg ml −1 cycloheximide). The cells were broken with glass beads and the cleared extract (OD 254 =5.0) was loaded on a 10.5 ml 5–45% sucrose gradient in extraction buffer lacking cycloheximide. Following centrifugation (16 h; 21,000 r.p.m. ; SW41 Beckman rotor), gradients were collected at a 1 ml min −1 flow rate and the ultraviolet profile recorded at 254 nm by a ultraviolet detector (linked to BioLogic LB fractionator), visualized with LP Data View software (Bio-Rad) and exported to Excel (Microsoft Office). For global translation analysis, cells were grown as described above. The cells were collected at an OD 600 =0.5 and washed with complete synthetic medium lacking methionine but containing 2% raffinose or 2% galactose. The cells were then resuspended in 1 ml of the corresponding medium and pulse-labelled with 100 μCi of 5′,6′ [ 3 H]- L -methionine for 20 min at 23 °C. Total proteins (TCA insoluble fraction) were extracted and washed twice with cold acetone before resolubilization. The amount of newly synthesized proteins was quantified using a scintillation counter. The solubilized proteins were also separated on a Nu-PAGE 4–10% gradient gel and Coomassie stained to evidence equal loading. For northern hybridization analysis, total RNA was isolated from the whole-cell extracts submitted to ribosome profiling (see above). Denaturing agarose gel electrophoresis, transferring of the RNA onto a positive membrane and northern hybridization with 32 P-labelled oligomers ( Supplementary Table 3 ) were performed as described [12] . In vitro phosphorylation of Rpa43 by Rio1 Recombinant Rpa43-His6-HA was produced in E. coli Rosetta BL21(DE3) cells. Expression of Rpa43-His6-HA from plasmid pRSET-43A (gift from M. Riva) was induced at an OD 600 =0.5 with 150 mM IPTG (3.5 h, 24 °C). Cells were collected in lysis buffer (20 mM Tris-Cl, pH8.0, 300 mM NaCl, 10% glycerol, 20 mM imidazole, 1 mM PMSF and 1 mM Na 3 VO 4 ) and lysed with a French press (15,000 p.s.i. ; Microfluidics). The extract was incubated with Ni 2+ -NTA beads (Qiagen). The beads were washed with 30 mM imidazole and Rpa43-His6-HA eluted with 200 mM imidazole before being submitted to size-exclusion chromatography (Superdex 200 HR 10/30, GE Healthcare). Recombinant His6-Rio1 was produced in E. coli BL21-RIL cells and expressed from plasmid pQE32-HIS6-RIO1 (gift from M. Angermayr) [21] . Expression was induced (3.5 h 30 °C) at an OD 600 =0.7 with 1 mM IPTG and the cells were collected in lysis buffer (50 mM NaH 2 PO 4 pH8.0, 50% glycerol, 300 mM NaCl, 1 mM NaF, 1 mM PMSF, 1 mM Na 3 VO 4 , 1 μg ml −1 apoprotein and leupeptine, 1 mg ml −1 lysozyme, 5 μg ml −1 DNase and 100 μg ml −1 RNAse). The cell extract, obtained with a French press, was incubated with Ni 2+ -NTA beads (Qiagen), which were then washed with 20 mM imidazole. His6-Rio1 was eluted with 200 mM imidazole and the buffer was then exchanged into 50 mM HEPES, pH7.5, 5% glycerol, 1 μg ml −1 apoprotein and leupeptine using PD-10 columns (GE Healthcare). The purity of Rpa43-His6-HA and His6-Rio1 was confirmed via SDS–PAGE and GelCode Blue (Pierce) staining. To examine phosphorylation of Rpa43-His6-HA by His6-Rio1, 1 μg of His6-Rio1, 6 μg of Rpa43-His6-HA and 0.05 μM (5 μCi) [γ- 32 P]ATP (PerkinElmer) were incubated (2 h, 30 °C) in reaction buffer (50 mM HEPES-KOH, pH 7.2, 5 mM MgCl 2 and 5 mM MnCl 2 ). Phosphorylated Rpa43-His6-HA was visualized radiographically. In the control reactions, only His6-Rio1 or Rpa43-His6-HA was present. To produce phosphorylated Rpa43-His6-HA for mass spectrometric analysis, five kinase reactions were set up, pooled (giving 30 μg Rpa43-His6-HA) and separated by SDS–PAGE. Proteins were stained with GelCode Blue, Rpa43-His6-HA then excised from the gel, submitted to proteolytic cleavage and analysed by nanoLC-MS/MS (see below). In the negative-control assay, ATP was omitted from the kinase reaction. NanoLC-MS/MS and data analysis The nano HPLC system was comprised of an UltiMate 3000 HPLC RSLC nano system (Thermo Fisher Scientific) coupled to a Q Exactive mass spectrometer (Thermo Fisher Scientific), equipped with a Proxeon nanospray source (Thermo Fisher Scientific). Following proteolytic treatment of Rpa43-His6-HA, peptides were loaded onto a trap column (PepMap C18, 5 mm × 300 μm ID, 5 μm particles, 100 Å pores; Thermo Fisher Scientific) at a flow rate of 25 μl min −1 using 0.1% TFA as mobile phase. After 10 min, the trap column was switched in line with the analytical column (PepMap C18, 500 mm × 75 μm ID, 3 μm, 100 Å; Thermo Fisher Scientific). The peptides were eluted using a flow rate of 230 nl min −1 , and a binary 2-h gradient and a 165-min gradient. The gradient starts with the mobile phases: 98% A (water/formic acid, 99.9/0.1, v/v) and 2% B (water/acetonitrile/formic acid, 19.92/80/0.08, v/v/v) increases to 35% B over the next 120 min, followed by a gradient in 5 min to 90% B, stays there for 5 min and decreases in 5 min back to the gradient 98% A and 2% B for equilibration at 30 °C. The Q Exactive mass spectrometer was operated in data-dependent mode, using a full scan ( m/z range 380–1,650, nominal resolution of 70,000; target value 3E6) followed by MS/MS scans of the 12 most abundant ions. MS/MS spectra were acquired using normalized collision energy 27%, isolation width of 2 and the target value was set to 1E5. Precursor ions selected for fragmentation (charge state 2 and higher) were put on a dynamic exclusion list for 10 s. In addition, the underfill ratio was set to 20% resulting in an intensity threshold of 4E4. The peptide match feature and the exclude isotopes feature were enabled. For peptide identification, the RAW files were loaded into Proteome Discoverer (version 1.4.0.288, Thermo Scientific). The created MS/MS spectra were searched using Mascot 2.2.07 (Matrix Science, Sequest, Thermo Scientific) [68] and MSAmanda [69] against the S. cerevisiae genome database [25] . The following search parameters were used: β-methylthiolation on cysteine was set as a fixed modification, mono- and dioxidation on methionine, acetylation on lysine and protein-N terminus, deamidation on asparagine and glutamine, mono- and dimethylation on lysine, and arginine and phosphorylation on serine, threonine and tyrosine were set as variable modifications. Monoisotopic masses were searched within unrestricted protein masses for tryptic and chymotryptic peptides. The peptide mass tolerance was set to ±6 ppm and the fragment mass tolerance to ±30 mmu. The maximal number of missed cleavages was set to 2. The result was filtered to 1% false discovery rate using the Percolator algorithm integrated in Proteome Discoverer (Thermo Scientific). The localization of the phosphorylation sites within the peptides was performed with ptmRS, based on the algorithm of phosphoRS [70] . The ion series of the Rpa43 QHLNPLVMKYNNK phospho-peptide are shown in Supplementary Table 4 . How to cite this article: Iacovella, M. G. et al. Rio1 promotes rDNA stability and downregulates RNA polymerase I to ensure rDNA segregation. Nat. Commun. 6:6643 doi: 10.1038/ncomms7643 (2015).